Light and pheromone-sensing neurons regulates cold habituation through insulin signalling inCaenorhabditis elegans Temperature is a critical environmental stimulus that has a strong impact on an organism’s biochemistry. Animals can respond to changes in ambient temperature through behaviour or altered physiology. However, how animals habituate to temperature is poorly understood. The nematode C. elegans stores temperature experiences and can induce temperature habituation-linked cold tolerance. Here we show that light and pheromone-sensing neurons (ASJ) regulate cold habituation through insulin signalling. Calcium imaging reveals that ASJ neurons respond to temperature. Cold habituation is abnormal in a mutant with impaired cGMP signalling in ASJ neurons. Insulin released from ASJ neurons is received by the intestine and neurons regulating gene expression for cold habituation. Thus, temperature sensation in a light and pheromone-sensing neuron produces a robust effect on insulin signalling that controls experience-dependent temperature habituation. Temperature is one of the most critical environmental stimuli and causes biochemical changes in the body. Animals including humans can, therefore, respond and habituate to changes in ambient temperature. The nematode Caenorhabditis elegans is a useful model for studying the mechanism of temperature habituation, because of its powerful molecular genetics. Previous study by Murray et al . [1] demonstrated that C. elegans has a cold tolerance that is regulated by phospholipid saturation. Savory et al . [2] previously reported that cold tolerance is regulated by molecules involved in the ageing pathway, such as FOXO-type transcription factors and PI3 kinase. The essential organs and tissues for systematic regulation of cold tolerance in C. elegans , however, remain unknown. In this study, we investigated the molecular physiological mechanisms underlying temperature experience-dependent cold tolerance in C. elegans . Our Ca 2+ imaging and genetic analyses reveal that light and pheromone-sensing (ASJ) neurons receive temperature input and transmit information through a photo signal-transduction pathway. Insulin released from ASJ neurons is received in the intestine and neurons, which controls cold habituation. Our study describes systematic regulation of cold habituation in a living animal. As previously reported by Murray et al . [1] and Savory et al . [2] , C. elegans has a cultivation temperature-dependent cold tolerance. Wild-type animals cultivated at 20 or 25 °C were killed by cold shock. In contrast, most wild-type animals cultivated at 15 °C survived after cold shock ( Fig. 1a ). To examine the conditions of temperature experience-dependent cold tolerance in detail, we used varying cold-shock temperatures (0–4 °C) ( Fig. 1b ), cultivation temperatures (13–27 °C) ( Fig. 1c ) and cold-shock times (6–240 h) ( Supplementary Fig. 1a–c ). Cold tolerance decreased when cultivation temperature was higher, when cold-shock temperature was lower and when cold-shock time was longer. We used 2 °C for 48 h as a typical cold-shock treatment for the majority of the following experiments. To determine whether cold tolerance was established at a specific developmental stage, we performed temperature shift experiments using larvae between the L1 and L4 stages ( Fig. 1d,e ). We found that a shift of cultivation temperature at larval stages did not severely affect the cold tolerance of adult animals ( Fig. 1d,e ). To understand how long it takes for cold tolerance to be established in adult animals, we shifted the temperature of adult animals ( Fig. 1f,g ). Unexpectedly, cold tolerance was established only 2–3 h after the cultivation temperature was changed from 25 to 15 °C ( Fig. 1f ) or from 20 to 15 °C ( Fig. 1g ). Furthermore, cold tolerance was diminished 2–3 h after the cultivation temperature was changed from 15 to 25 °C ( Supplementary Fig. 1d ) or 20 to 25 °C ( Supplementary Fig. 1e ). 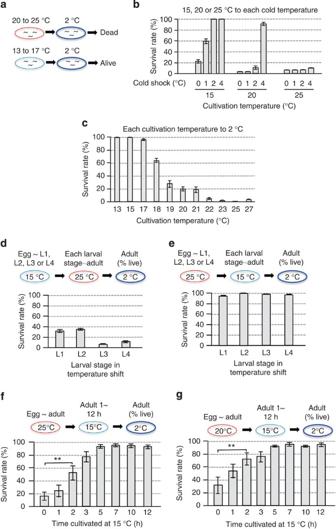Figure 1: Temperature experience-inducing cold tolerance phenotype in wild type. N2 (Bristol) strain was used as the wild-type animal in all experiments for this figure. (a) Cultivation temperature-dependent cold tolerance. Twenty to twenty-five degree centigrade-cultivated animals cannot live after cultivation at 2 °C for 48 h, while 13–17 °C-cultivated animals can live after 48 h at 2 °C. (b) Effect of cold-shock temperatures (0, 1, 2 and 4 °C). Fifteen degree centigrade-cultivated animals can survive at 2 and 4 °C. Twenty degree centigrade-cultivated animals can survive at 4 °C. Twenty-five degree centigrade-cultivated animals cannot survive at 0–4 °C. For each assay,n≥6. (c) Effect of cultivation temperatures (from 13–27 °C). Thirteen to fifteen degree centigrade-cultivated animals can survive at 2 °C, while 20–27 °C-cultivated animals cannot survive at 2 °C. For each assay,n≥6. (d,e) Temperature shift experiments using L1 to L4 stage larvae (15–25 °C (d) or 25–15 °C (e)). Worms are initially cultivated at the first temperature (15 °C (d) or 25 °C (e)) from egg to each larval stage, and then worms were transferred to the second temperature (25 °C (d) or 15 °C (e)) and cultivated until they reached adult stage. After the adult worms were subjected to cold shock (2 °C, 48 h), survival rate was calculated. Cold tolerance is not dependent on the temperature experience at the larval stage. For each assay,n≥6. (f,g) Temperature shift experiments at the adult stage (25–15 °C (f) or 20–15 °C (g)). Worms were cultivated at the first temperature (25 °C (f) or 20 °C (g)) until they reached the adult stage, and then worms were transferred to the second temperature (15 °C (f,g)) and cultivated for specific times (0–12 h indicated on the horizontal axis). After the temperature shifted-adult worms were subjected to cold shock (2 °C, 48 h), survival rate was calculated. About 3 h after the cultivation temperature was changed, cold tolerance was acquired. For each assay,n≥6. Error bars indicate standard error of the mean. analysis of variance followed by Dunnetpost-hoctest was used for multiple comparisons. **P<0.01. Detailed-phenotypic analyses indicated that temperature experience for the formation of cold tolerance can be overwritten within 2–3 h. Figure 1: Temperature experience-inducing cold tolerance phenotype in wild type. N2 (Bristol) strain was used as the wild-type animal in all experiments for this figure. ( a ) Cultivation temperature-dependent cold tolerance. Twenty to twenty-five degree centigrade-cultivated animals cannot live after cultivation at 2 °C for 48 h, while 13–17 °C-cultivated animals can live after 48 h at 2 °C. ( b ) Effect of cold-shock temperatures (0, 1, 2 and 4 °C). Fifteen degree centigrade-cultivated animals can survive at 2 and 4 °C. Twenty degree centigrade-cultivated animals can survive at 4 °C. Twenty-five degree centigrade-cultivated animals cannot survive at 0–4 °C. For each assay, n ≥6. ( c ) Effect of cultivation temperatures (from 13–27 °C). Thirteen to fifteen degree centigrade-cultivated animals can survive at 2 °C, while 20–27 °C-cultivated animals cannot survive at 2 °C. For each assay, n ≥6. ( d , e ) Temperature shift experiments using L1 to L4 stage larvae (15–25 °C ( d ) or 25–15 °C ( e )). Worms are initially cultivated at the first temperature (15 °C ( d ) or 25 °C ( e )) from egg to each larval stage, and then worms were transferred to the second temperature (25 °C ( d ) or 15 °C ( e )) and cultivated until they reached adult stage. After the adult worms were subjected to cold shock (2 °C, 48 h), survival rate was calculated. Cold tolerance is not dependent on the temperature experience at the larval stage. For each assay, n ≥6. ( f , g ) Temperature shift experiments at the adult stage (25–15 °C ( f ) or 20–15 °C ( g )). Worms were cultivated at the first temperature (25 °C ( f ) or 20 °C ( g )) until they reached the adult stage, and then worms were transferred to the second temperature (15 °C ( f , g )) and cultivated for specific times (0–12 h indicated on the horizontal axis). After the temperature shifted-adult worms were subjected to cold shock (2 °C, 48 h), survival rate was calculated. About 3 h after the cultivation temperature was changed, cold tolerance was acquired. For each assay, n ≥6. Error bars indicate standard error of the mean. analysis of variance followed by Dunnet post-hoc test was used for multiple comparisons. ** P <0.01. Full size image We next investigated which tissues were involved in temperature experience-dependent cold tolerance, by examining the phenotypes of various tissue-specific mutants. We found that a mutant with defective unc-104 /kinesin in almost all neurons showed abnormal enhancement of cold tolerance after cultivation at 20 °C ( Fig. 2a ) [3] , [4] . By contrast, mutants with impairments in the cuticle or body wall muscle did not display cold tolerance abnormalities ( Fig. 2a ). These data suggest that temperature experience-dependent cold tolerance is regulated, at least in part, by neurons. A known-neural circuit for thermotaxis behaviour of C. elegans involves temperature sensing and processing [5] , [6] . We next examined the cold tolerance of mutants defective in the development or function of the temperature-sensing neurons participating in the thermotaxis neural circuit, AFD and AWC, and their downstream interneurons AIY and RIA ( Fig. 2b ; Supplementary Fig. 2a ) [5] , [6] , [7] . Developmental or functional defects of these component neurons of the thermotaxis circuit did not lead to abnormal cold tolerance ( Fig. 2b ), suggesting that this known temperature-processing neural circuit is not essential for temperature experience-dependent cold tolerance. We found that the thermotaxis mutant, tax-6 , which lacks calcineurin function in many neurons, had abnormal cold tolerance ( Fig. 2b ) [8] , [9] . This abnormality was partially rescued by the expression of the tax-6 gene in sensory neurons as well as in almost all neurons ( Fig. 2b , tax-6;Ex[unc-14p:: tax-6] (almost all neurons), tax-6;Ex[tax-6p (1.1 kb) ::tax-6] (many sensory neurons (amphid and phasmid))). These results imply that sensory neurons are important for cold tolerance. We therefore measured temperature experience-dependent cold tolerance in mutants with defective sensory neurons ( Fig. 2c ; Supplementary Fig. 2b ). Mutant animals with impaired che-13 and osm-6 genes demonstrated severely abnormal cold tolerance after cultivation at 20 °C ( Fig. 2c ). Both che-13 and osm-6 genes encode components of an intraflagellar transport complex that is essential for cilium function in the sensory ending of sensory neurons ( Supplementary Fig. 2b ) [10] , [11] , [12] , [13] , suggesting that sensory input may be essential for cold tolerance. 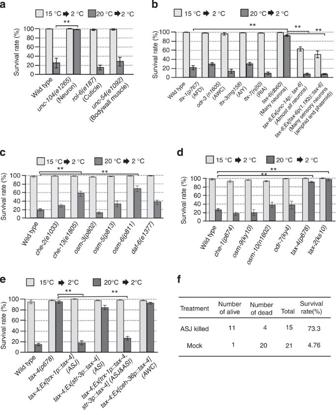Figure 2: ASJ sensory neurons are essential for cold tolerance. (a) Mutants impairing specific tissue functions. Mutant impairingunc-104/kinesin expression in neurons showed abnormal cold tolerance after cultivation at 20 °C, whereas mutants impairingrol-6/cuticle orunc-54/muscles did not show the defect. Strain names and alleles are indicated. For each assay,n≥6. (b) Mutants showing developmental or functional defects in thermotaxis neurons, AFD, AWC, AIY and RIA, did not demonstrate abnormal cold tolerance.tax-6mutants showed abnormal cold tolerance, which was partially rescued by expressing thetax-6gene in all neurons (unc-14p::tax-6) or in sensory neurons (tax-6p(1.1 kb)::tax-6)8. The detailed information of these promoters is indicated in the Methods section. For each assay,n≥6. (c,d) Cold tolerance of mutants affecting sensory neurons. Gene products and cells expressing each gene are listed inSupplementary Fig. 2b. Bothche-13andosm-6mutants showed abnormal increments of cold tolerance after 20 °C cultivation (c). Twenty degree centigrade-cultivatedtax-4andtax-2mutants, encoding the cGMP-gated channel, showed significant increments in cold tolerance (d). For each assay,n≥6. (e) Cell-specific expression oftax-4 cDNAintax-4(p678) mutants. The promoters for cell-specific expression used in this experiment were thetrx-1promoter (ASJ),str-3promoter (ASI) andceh-36promoter (AWC). Abnormal cold tolerance intax-4(p678)was rescued by specific expression oftax-4 cDNAin ASJ sensory neurons. For each assay,n≥6. (f) Laser-killing of ASJ sensory neurons affects normal cold tolerance. ASJ-ablated wild-type animals showed abnormal cold tolerance phenotypes after 20 °C cultivation. The survival rate of ASJ-ablated animals was significantly increased from that of mock-treated wild-type animals. Error bars indicate standard error of the mean. analysis of variance followed by Dunnetpost-hoctest was used for multiple comparisons. **P<0.01. Figure 2: ASJ sensory neurons are essential for cold tolerance. ( a ) Mutants impairing specific tissue functions. Mutant impairing unc-104 /kinesin expression in neurons showed abnormal cold tolerance after cultivation at 20 °C, whereas mutants impairing rol-6 /cuticle or unc-54 /muscles did not show the defect. Strain names and alleles are indicated. For each assay, n ≥6. ( b ) Mutants showing developmental or functional defects in thermotaxis neurons, AFD, AWC, AIY and RIA, did not demonstrate abnormal cold tolerance. tax-6 mutants showed abnormal cold tolerance, which was partially rescued by expressing the tax-6 gene in all neurons ( unc-14p::tax-6 ) or in sensory neurons ( tax-6p (1.1 kb) ::tax-6 ) [8] . The detailed information of these promoters is indicated in the Methods section. For each assay, n ≥6. ( c , d ) Cold tolerance of mutants affecting sensory neurons. Gene products and cells expressing each gene are listed in Supplementary Fig. 2b . Both che-13 and osm-6 mutants showed abnormal increments of cold tolerance after 20 °C cultivation (c). Twenty degree centigrade-cultivated tax-4 and tax-2 mutants, encoding the cGMP-gated channel, showed significant increments in cold tolerance ( d ). For each assay, n ≥6. ( e ) Cell-specific expression of tax-4 cDNA in tax-4(p678 ) mutants. The promoters for cell-specific expression used in this experiment were the trx-1 promoter (ASJ), str-3 promoter (ASI) and ceh-36 promoter (AWC). Abnormal cold tolerance in tax-4(p678) was rescued by specific expression of tax-4 cDNA in ASJ sensory neurons. For each assay, n ≥6. ( f ) Laser-killing of ASJ sensory neurons affects normal cold tolerance. ASJ-ablated wild-type animals showed abnormal cold tolerance phenotypes after 20 °C cultivation. The survival rate of ASJ-ablated animals was significantly increased from that of mock-treated wild-type animals. Error bars indicate standard error of the mean. analysis of variance followed by Dunnet post-hoc test was used for multiple comparisons. ** P <0.01. Full size image To identify essential sensory neurons for temperature experience-dependent cold tolerance ( Fig. 2d ; Supplementary Fig. 2b ), we tested the cold tolerance of mutants defective in specific or multiple sensory neurons. A strong abnormality was observed in tax-4 and tax-2 mutants lacking cGMP-gated channels that are expressed in several sensory neurons, such as AFD, AWC, ASJ and ASI ( Fig. 2d ; Supplementary Fig. 2b ) [14] . We therefore expressed tax-4 complementary DNA (cDNA) in ASJ, AWC and/or ASI sensory neurons of tax-4 mutants using cell-specific promoters ( Fig. 2e , tax-4;Ex[trx-1p::tax-4] (ASJ), tax-4;Ex[str-3p::tax-4] (ASI) and tax-4;Ex[ceh-36p::tax-4] (AWC)) . We found that the abnormality of tax-4 mutants was rescued by the specific expression of tax-4 cDNA in a single pair of sensory neurons, ASJ neurons, which are known as light and pheromone-sensing neurons ( Fig. 2e ) [15] . In addition, laser ablation of ASJ sensory neurons in wild-type animals induced abnormal cold tolerance, which was similar to the tax-4 mutant phenotype ( Fig. 2f ). These results suggest that cultivation temperature-dependent cold tolerance is controlled by ASJ sensory neurons, and that ASJ neurons negatively regulate cold tolerance. We hypothesized that ASJ neurons act as thermosensory neurons. To examine this hypothesis, we used the genetically encoded calcium indicator, cameleon [16] , [17] , to perform calcium imaging of the ASJ neuron under temperature changes. The cameleon gene, yc3.60 , was expressed in ASJ sensory neurons under the trx-1 promoter. We found that the calcium concentration in ASJ neurons changes in response to temperature ( Fig. 3a,b ; Supplementary Fig. 2c,d ). By contrast, this temperature response was decreased in the tax-4 mutant, which lacks a cGMP-gated channel essential for sensory signalling in ASJ ( Fig. 3c,d ). The defect in tax-4 mutants was rescued by specific expression of tax-4 cDNA in ASJ neurons, even in the absence of expression in the sensory neurons that regulate thermotaxis, such as AFD, AWC and ASI ( Fig. 3c,d ). Thus, physiological and genetic analyses suggest that ASJ acts as a temperature-sensing neuron. Moreover, the temperature response of ASJ was normal in the mutant with impaired SNB-1/synaptobrevin ( Fig. 3f ), suggesting that ASJ responses to temperature changes are cell autonomous and do not require neurochemical input from other neurons. 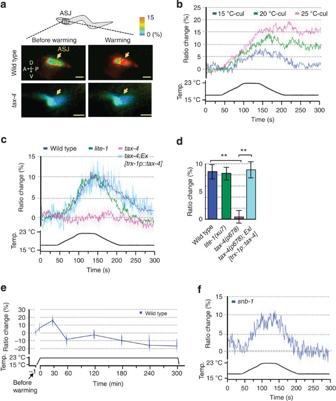Figure 3: Neural activity of ASJ sensory neuron with temperature stimuli. (a) Wild type and mutant expressing yellow cameleon driven bytrx-1promoter,trx-1p::yc3.60(pTOM13), were tested by calcium imaging. Representative fluorescence resonance energy transfer signal in ASJ of wild type ortax-4mutant cultivated at 15 °C when worms were subjected to temperature changes. A schematic diagram of an ASJ in head, and corresponding pseudo colour images depicting fluorescence ratio of cameleon before and during temperature change. Arrows, indicate ASJ cell body. Scale bar, 10 μm. (b,c,f)In vivocalcium imaging of ASJ from wild type cultivated at each temperature (b), mutants (c,f). Relative increase or decrease in the intracellular Ca2+concentration was measured as an increase or decrease in yellow fluorescent protein/cyan fluorescent proteins fluorescence ratio of the cameleon (ratio change) during temperature changes. Temperature changes (ranging from 17–23 °C) with time are shown at the bottom of the graph. Calcium concentrations in ASJ of wild type change following temperature stimuli, which were observed in animals cultivated at different temperatures (b). Calcium concentration changes responding to temperature shifts were not observed intax-4(p678)(c).lite-1andtax-4;Ex[trx-1p::tax-4], which isa tax-4mutant with specifically expressingtax-4 cDNAin ASJ, could respond to temperature changes (c).snb-1 (md247)mutants also responded (f). Each graph represents average response to temperature stimuli (b,c,f).n=12–17. (d) Bar graph showing average ratio change during 20 s from 120 to 140 s of the experiment indicated in (c). Colour key for bar graph is the same as that for the corresponding response curve in (c). (e) Calcium imaging of ASJ in wild type during longer times. At 30 min after temperature shift, intracellular Ca2+concentration in ASJ was at its maximum, after which a decrease was observed and stabilized. Fluorescence ratio was measured at −1, 0, 30, 60, 120, 180, 240 and 300 min after temperature change. At each time point, fluorescence signal of cameleon was detected for 60 s. Two Scale bars, −1 to 0 min and 0 to 300 min, are shown on the horizontal line. The data were sequentially measured in chronological order using individual animals.n=13. Error bars indicate standard error of the mean. Analysis of variance followed by Dunnetpost-hoctest was used for multiple comparisons. **P<0.01. Figure 3: Neural activity of ASJ sensory neuron with temperature stimuli. ( a ) Wild type and mutant expressing yellow cameleon driven by trx-1 promoter, trx-1p::yc3.60 (pTOM13), were tested by calcium imaging. Representative fluorescence resonance energy transfer signal in ASJ of wild type or tax-4 mutant cultivated at 15 °C when worms were subjected to temperature changes. A schematic diagram of an ASJ in head, and corresponding pseudo colour images depicting fluorescence ratio of cameleon before and during temperature change. Arrows, indicate ASJ cell body. Scale bar, 10 μm. ( b , c , f ) In vivo calcium imaging of ASJ from wild type cultivated at each temperature ( b ), mutants ( c , f ). Relative increase or decrease in the intracellular Ca 2+ concentration was measured as an increase or decrease in yellow fluorescent protein/cyan fluorescent proteins fluorescence ratio of the cameleon (ratio change) during temperature changes. Temperature changes (ranging from 17–23 °C) with time are shown at the bottom of the graph. Calcium concentrations in ASJ of wild type change following temperature stimuli, which were observed in animals cultivated at different temperatures ( b ). Calcium concentration changes responding to temperature shifts were not observed in tax-4(p678) ( c ). lite-1 and tax-4 ; Ex[trx-1p::tax-4] , which is a tax-4 mutant with specifically expressing tax-4 cDNA in ASJ, could respond to temperature changes ( c ). snb-1 (md247) mutants also responded ( f ). Each graph represents average response to temperature stimuli ( b , c , f ). n =12–17. ( d ) Bar graph showing average ratio change during 20 s from 120 to 140 s of the experiment indicated in ( c ). Colour key for bar graph is the same as that for the corresponding response curve in ( c ). ( e ) Calcium imaging of ASJ in wild type during longer times. At 30 min after temperature shift, intracellular Ca 2+ concentration in ASJ was at its maximum, after which a decrease was observed and stabilized. Fluorescence ratio was measured at −1, 0, 30, 60, 120, 180, 240 and 300 min after temperature change. At each time point, fluorescence signal of cameleon was detected for 60 s. Two Scale bars, −1 to 0 min and 0 to 300 min, are shown on the horizontal line. The data were sequentially measured in chronological order using individual animals. n =13. Error bars indicate standard error of the mean. Analysis of variance followed by Dunnet post-hoc test was used for multiple comparisons. ** P <0.01. Full size image To analyze whether acclimation temperature alters ASJ neuron responsiveness to the temperature stimulus, we monitored calcium concentration changes in ASJ neurons of wild-type animals that were cultivated at 15, 20 or 25 °C, by calcium imaging. Physiological analysis in this study suggested that the temperature response of ASJ neurons is altered by the cultivation temperature ( Fig. 3b ). We found that calcium concentration changes in ASJ neurons of 20 or 25-°C-cultivated animals were stronger than those of 15-°C-cultivated animals. These results are consistent with the genetic results in this study that ASJ neurons negatively regulate cold tolerance, where reduced-ASJ activity enhances cold tolerance and increased-ASJ activity reduces cold tolerance. To determine what molecules are involved in temperature signalling in ASJ neurons, we tested mutants defective in phototransduction in ASJ neurons [15] . We found that mutants of proteins involved in phototransduction in ASJ neurons, including trimeric G protein alpha subunits ( gpa-1, gpa-3 or goa-1) , guanylyl cyclase ( daf-11; odr-1 ) or phosphodiesterase ( pde-1; pde-2 ), showed abnormalities in cold tolerance ( Fig. 4a,b ). Although the specific neuron responsible for these abnormalities in cold tolerance was not determined, these results are consistent with a hypothesis that two sensory modalities, light and temperature, are transduced by shared signalling molecules. A lite-1 mutant, lacking a photoreceptor protein expressed in ASJ neurons, showed normal cold tolerance ( Fig. 4a,b ) and normal calcium concentration changes in ASJ neurons in response to temperature changes ( Fig. 3c ) [15] . Therefore, temperature is probably received in ASJ neurons by other receptors. 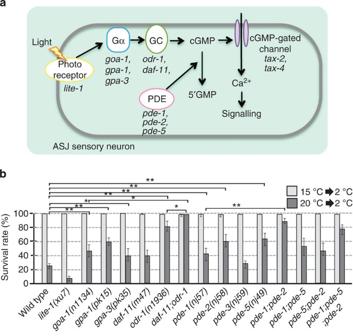Figure 4: Temperature information is processed through the cGMP pathway in ASJ neurons. (a) A molecular model of phototransduction in ASJ neurons, which is mediated by trimeric G-proteins and cGMP-dependent signalling15. (b) Cold tolerance of mutants with an impaired light-sensing pathway in ASJ neurons, which contains photoreceptor (lite-1), trimeric G protein alpha subunits (goa-1, gpa-1andgpa-3), guanylyl cyclase (daf-11andodr-1) and phosphodiesterase (pde-1to5). Allele names of double or triple mutants are the same for each single mutant. For each assay,n≥6. Error bars indicate standard error of the mean. Analysis of variance followed by Dunnetpost-hoctest was used for multiple comparisons. *P<0.05; **P<0.01. Abbreviations: cGMP, cyclic guanosine monophosphate; Gα, trimeric G protein alpha subunit; GC, guanylyl cyclase; PDE, phosphodiesterase. Figure 4: Temperature information is processed through the cGMP pathway in ASJ neurons. ( a ) A molecular model of phototransduction in ASJ neurons, which is mediated by trimeric G-proteins and cGMP-dependent signalling [15] . ( b ) Cold tolerance of mutants with an impaired light-sensing pathway in ASJ neurons, which contains photoreceptor ( lite-1 ), trimeric G protein alpha subunits ( goa-1, gpa-1 and gpa-3) , guanylyl cyclase ( daf-11 and odr-1 ) and phosphodiesterase ( pde-1 to 5 ). Allele names of double or triple mutants are the same for each single mutant. For each assay, n ≥6. Error bars indicate standard error of the mean. Analysis of variance followed by Dunnet post-hoc test was used for multiple comparisons. * P <0.05; ** P <0.01. Abbreviations: cGMP, cyclic guanosine monophosphate; Gα, trimeric G protein alpha subunit; GC, guanylyl cyclase; PDE, phosphodiesterase. Full size image We next investigated how ASJ sensory neurons control temperature experience-dependent cold tolerance. We demonstrated that mutants defective in synaptic transmission, including mutants of SNB-1/Synaptobrevin, SNT-1/Synaptotagmin, UNC-64/Syntaxin or EGL-21/Neuropeptide processing enzyme, showed abnormal enhancement of cold tolerance phenotypes that were similar to those of ASJ-defective mutants ( Fig. 5a ). These results imply that neurotransmission is important for cold tolerance. 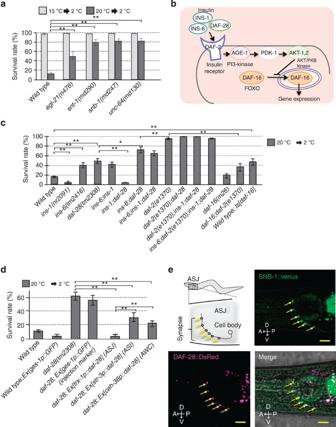Figure 5: Insulin signalling is involved in cold tolerance. (a) Cold tolerance of mutants with impaired synaptic transmission containing carboxypeptidase (egl-21), synaptotagmin (snt-1), synaptobrevin (snb-1) and syntaxin(unc-64). These mutants showed abnormal increments in cold tolerance. For each assay,n≥6. (b) A model of insulin signalling in dauer formation based on previous reports23,24,27.ins-1, ins-6anddaf-28encode insulin.daf-2encodes the insulin receptor only inC. elegans.age-1 and pdk-1encode phosphoinositide 3-kinase and 3-phosphoinositide dependent kinase, respectively.akt-1andakt-2encode serine/threonine kinase.daf-16encodes FOXO transcription factor. Downstream cascade of DAF-2/insulin receptor contains AGE-1, PDK-1, AKT-1 and AKT-2. AKT-1 and AKT-2 inhibit nuclear translocation of DAF-16. Therefore, DAF-2 signalling negatively regulates DAF-16 in dauer formation. (c) Cold tolerance of mutants defective in insulin signalling. Animals of all strains were cultivated at 15 °C from egg to L4 larvae, and after that, animals were cultivated at 20 °C overnight from L4 to adult, because many insulin-signalling mutants showed constitutive dauer formation (daf-c) at 20 °C. Wild type; Is[daf-16]is an N2 strain with an integrated form of DAF-16::GFP, which also showsdaf-c46. For each assay,n≥9. (d) Cell-specific rescue experiments ofdaf-28null mutants. Cell-specific promoters used in this experiment weretrx-1,str-3orceh-36promoters for expression in ASJ, ASI or AWC cells, respectively.ges-1p::NLS-GFPwas co-injected as a transgenic marker in all transgenic strains. For each assay,n≥9. (e) Localization of DAF-28 at the synapse of ASJ. Wild type with ASJ-specific expression of DAF-28::dsRedm and SNB-1::VENUS (wild type;Ex[trx-1p::daf-28::dsRedm, trx-1p::snb-1::VENUS]) were analyzed by confocal microscopy. The upper-left panel indicates a schematic diagram of synapses in ASJ of head. In the upper-right panel, arrows indicate localization of synaptobrevin (SNB-1)::VENUS at synapses in ASJ. In the bottom-left panel, arrows indicate localization of DAF-28::dsRedm in ASJ. The bottom-right panel is the merged image of upper-right panel, bottom-left panel and bright-field image. In the merged image, arrows indicate white regions that suggest co-localization of SNB-1::VENUS and DAF-28::DsRedm at synapses. Scale bar, 10 μm. Error bars indicate standard error of the mean. Analysis of variance followed by Dunnetpost-hoctest was used for multiple comparisons. *P<0.05; **P<0.01. Figure 5: Insulin signalling is involved in cold tolerance. ( a ) Cold tolerance of mutants with impaired synaptic transmission containing carboxypeptidase ( egl-21 ), synaptotagmin ( snt-1 ), synaptobrevin ( snb-1 ) and syntaxin (unc-64 ). These mutants showed abnormal increments in cold tolerance. For each assay, n ≥6. ( b ) A model of insulin signalling in dauer formation based on previous reports [23] , [24] , [27] . ins-1, ins-6 and daf-28 encode insulin. daf-2 encodes the insulin receptor only in C. elegans . age-1 and pdk-1 encode phosphoinositide 3-kinase and 3-phosphoinositide dependent kinase, respectively. akt-1 and akt-2 encode serine/threonine kinase. daf-16 encodes FOXO transcription factor. Downstream cascade of DAF-2/insulin receptor contains AGE-1, PDK-1, AKT-1 and AKT-2. AKT-1 and AKT-2 inhibit nuclear translocation of DAF-16. Therefore, DAF-2 signalling negatively regulates DAF-16 in dauer formation. ( c ) Cold tolerance of mutants defective in insulin signalling. Animals of all strains were cultivated at 15 °C from egg to L4 larvae, and after that, animals were cultivated at 20 °C overnight from L4 to adult, because many insulin-signalling mutants showed constitutive dauer formation ( daf-c ) at 20 °C. Wild type ; Is[daf-16] is an N2 strain with an integrated form of DAF-16::GFP, which also shows daf-c [46] . For each assay, n ≥9. ( d ) Cell-specific rescue experiments of daf-28 null mutants. Cell-specific promoters used in this experiment were trx-1 , str-3 or ceh-36 promoters for expression in ASJ, ASI or AWC cells, respectively. ges-1p::NLS-GFP was co-injected as a transgenic marker in all transgenic strains. For each assay, n ≥9. ( e ) Localization of DAF-28 at the synapse of ASJ. Wild type with ASJ-specific expression of DAF-28::dsRedm and SNB-1::VENUS (wild type; Ex[trx-1p::daf-28::dsRedm, trx-1p::snb-1::VENUS] ) were analyzed by confocal microscopy. The upper-left panel indicates a schematic diagram of synapses in ASJ of head. In the upper-right panel, arrows indicate localization of synaptobrevin (SNB-1)::VENUS at synapses in ASJ. In the bottom-left panel, arrows indicate localization of DAF-28::dsRedm in ASJ. The bottom-right panel is the merged image of upper-right panel, bottom-left panel and bright-field image. In the merged image, arrows indicate white regions that suggest co-localization of SNB-1::VENUS and DAF-28::DsRedm at synapses. Scale bar, 10 μm. Error bars indicate standard error of the mean. Analysis of variance followed by Dunnet post-hoc test was used for multiple comparisons. * P <0.05; ** P <0.01. Full size image Previous reports suggest that cold tolerance is mediated by insulin-signalling pathways that are similar to pathways involved in dauer larva formation and ageing, and other stress tolerances, including oxidative stress [18] , [19] , ultraviolet light [20] , heavy metals [21] and microbial infections [22] , [23] . However, specific insulin molecules and specific tissues involved in cold tolerance have not been determined. C. elegans has 40 genes encoding insulin-like molecules. We focused on two, DAF-28 and INS-6, which are expressed in ASJ sensory neurons [24] . We found that mutant animals defective in DAF-28 and INS-6 showed partial enhancement of cold tolerance ( Fig. 5b,c ; Supplementary Fig. 4c ). Expressing daf-28cDNA in ASJ neurons of daf-28 mutants rescued abnormal cold tolerance, while expressing daf-28cDNA in AWC neurons reduced the abnormality but tolerance did not return to wild-type levels ( Fig. 5d ). Previous reports demonstrated that AWC neurons probably act as a temperature-sensing neuron, and that the endogenous daf-28 gene is not expressed in AWC sensory neurons from wild-type animals [6] , [25] . Based on these data, DAF-28 could be released from AWC by temperature stimuli in wild-type animals ectopically expressing daf-28 in AWC. Because the endogenous daf-28 gene is not expressed in wild-type AWC sensory neurons, these results suggest that DAF-28/insulin acts in a non-cell autonomous way, and is partially dependent on the neuron type. Similarly, a non-cell autonomous phenomenon is observed in the secretory-signalling pathways of sensory neurons in C. elegans , such as insulin/INS-1-dependent temperature learning behaviour and neuropeptide-dependent neural discrimination [26] , [27] . In both cases, ectopic expression of secretory genes in sensory neurons of mutants partially rescued the abnormal phenotype of mutants. Localization analysis using fluorescent proteins indicated that DAF-28 was co-localized with SNB-1/synaptobrevin at the synaptic region in ASJ neurons ( Fig. 5e ). By contrast, abnormal localization of DAF-28 in the cell body was observed in ASJ neurons of mutants with impaired UNC-104/kinesin, which is essential for cold tolerance ( Supplementary Fig. 4d ). These results imply that DAF-28/insulin is released from the synaptic region, and that DAF-28 is transported by kinesin into the synapse. To determine the molecules downstream of insulin in temperature experience-dependent cold tolerance, we tested various mutants defective in the known insulin-signalling pathway ( Figs 5b,c and 6a ). Phenotypic analysis showed that mutants defective in the DAF-2/insulin receptor or its downstream molecules showed abnormal enhancement of cold tolerance ( Figs 5c and 6a ; Supplementary Fig. 4c ) [28] . These results are consistent with a previous report showing that AGE-1/PI3 kinase and DAF-16/FOXO are involved in cold tolerance [2] . DAF-2 is the only insulin receptor in C. elegans , while there are about 40 ligands for insulin receptors. Genetic epistasis analysis revealed that two insulins, DAF-28 and INS-6, are both positive agonists that work redundantly on the DAF-2/insulin receptor in cold tolerance, because an ins-6; daf-28 double mutant showed a stronger phenotype than each single mutant ( Fig. 5c ) [25] , [29] . Additional genetic epistasis analysis indicated that INS-1/insulin genetically inhibits the DAF-2/insulin receptor through a negative regulation of INS-6/insulin ( Fig. 5c , Supplementary Fig. 4c ) [26] , [30] . Abnormal increments of cold tolerance in daf-2 mutants were suppressed by mutation in the DAF-16/FOXO-type transcriptional factor ( Fig. 5c ). We found that daf-16 mutant animals showed reduced cold tolerance after cultivation at 18 °C ( Supplementary Fig. 4b ), although daf-16 mutant animals did not show decreased cold tolerance after cultivation at 20 or 15 °C ( Fig. 5c ; Supplementary Fig. 4a ). In contrast, overexpression of the daf-16 gene induced abnormal increments of cold tolerance ( Fig. 5c (wild type; Is[daf-16] )). These results suggest that DAF-2/insulin receptor signalling and DAF-16/FOXO act as negative and positive regulators for cold tolerance, respectively. Because 15 °C-cultivated mutant animals defective in insulin signalling appeared to be cold tolerant ( Supplementary Fig. 4a ), it is probable that additional signalling pathways exist that lead to cold tolerance. 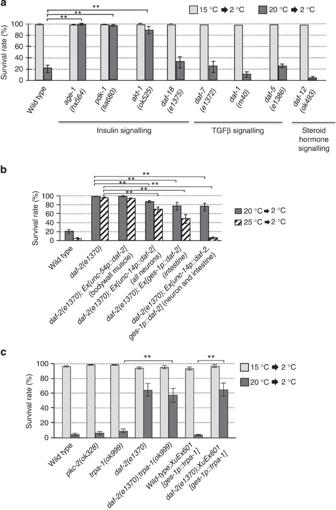Figure 6: Insulin signalling regulates gene expression during cold tolerance. (a) Temperature experience-dependent cold tolerance of mutants defective in insulin signalling, TGF-β signalling or steroid hormone signalling. Mutants defective in insulin signalling showed abnormal cold tolerance after 20 °C cultivation. In contrast, mutants of TGF-β signalling and steroid hormone signalling showed normal cold tolerance. For each assay,n≥6. (b) Tissue-specific rescue experiments ofdaf-2null mutants. For each assay,n≥9. Tissue-specific promoters used in this experiment were theunc-54promoter (body wall muscle),unc-14promoter (all neurons) andges-1promoter (intestine).ges-1p::daf-2cDNAandunc-14p::daf-2cDNAwere co-injected to allow co-expression in both the intestine and neurons. Abnormalities in 25 °C-cultivateddaf-2animals were rescued bydaf-2 cDNAco-expressed in both the intestine and neurons. For each assay,n≥9. (c) Cold tolerance in the cold receptor TRP channel and downstream signalling mutant33. PKC-2 is a downstream molecule of cold receptor/TRPA-1 that functions in the intestine.pkc-2andtrpa-1mutants did not show abnormal defects in cold tolerance. Thetrpa-1mutation did not affect cold tolerance in thedaf-2; trpa-1double mutant.daf-2; trpa-1, wild type; XuEx601anddaf-2(e1370); XuEx601strains were kindly provided by Dr Xu33. Overexpression of TRPA-1 also did not affect cold tolerance in both the wild type anddaf-2(e1370)mutant. For each assay,n≥9. Animals with thedaf-2(e1370)mutation were cultivated at 15 °C from egg to L4 larvae, and after that, animals were cultivated at 20 or 25 °C overnight from L4 to adult because of thedaf-cphenotype (b,c). Error bars indicate standard error of the mean. Analysis of variance followed by Dunnetpost-hoctest was used for multiple comparisons. **P<0.01. Figure 6: Insulin signalling regulates gene expression during cold tolerance. ( a ) Temperature experience-dependent cold tolerance of mutants defective in insulin signalling, TGF-β signalling or steroid hormone signalling. Mutants defective in insulin signalling showed abnormal cold tolerance after 20 °C cultivation. In contrast, mutants of TGF-β signalling and steroid hormone signalling showed normal cold tolerance. For each assay, n ≥6. ( b ) Tissue-specific rescue experiments of daf-2 null mutants. For each assay, n ≥9. Tissue-specific promoters used in this experiment were the unc-54 promoter (body wall muscle), unc-14 promoter (all neurons) and ges-1 promoter (intestine). ges-1p::daf-2cDNA and unc-14p::daf-2cDNA were co-injected to allow co-expression in both the intestine and neurons. Abnormalities in 25 °C-cultivated daf-2 animals were rescued by daf-2 cDNA co-expressed in both the intestine and neurons. For each assay, n ≥9. ( c ) Cold tolerance in the cold receptor TRP channel and downstream signalling mutant [33] . PKC-2 is a downstream molecule of cold receptor/TRPA-1 that functions in the intestine. pkc-2 and trpa-1 mutants did not show abnormal defects in cold tolerance. The trpa-1 mutation did not affect cold tolerance in the daf-2; trpa-1 double mutant. daf-2; trpa-1 , wild type ; XuEx601 and daf-2(e1370); XuEx601 strains were kindly provided by Dr Xu [33] . Overexpression of TRPA-1 also did not affect cold tolerance in both the wild type and daf-2(e1370) mutant. For each assay, n ≥9. Animals with the daf-2(e1370) mutation were cultivated at 15 °C from egg to L4 larvae, and after that, animals were cultivated at 20 or 25 °C overnight from L4 to adult because of the daf-c phenotype ( b , c ). Error bars indicate standard error of the mean. Analysis of variance followed by Dunnet post-hoc test was used for multiple comparisons. ** P <0.01. Full size image As previously reported, mutations in the insulin pathway, including the daf-2 mutation, extend lifespan, which induce better tolerance under a variety of stress conditions. An ambient temperature of 2 °C is considered an extremely stressful environment for worms. We tested cold tolerance of the mutants, hsf-1 /heat-shock factor, jnk-1 /MAP kinase, kgb-1 and kgb-2 /MAP kinase, and hsp-16.2 , hsp-16.41 and hsp-16.48 /heat-shock proteins, which are involved in the stress response. Phenotypic analysis of cold tolerance of these mutants showed that these mutants had a phenotype similar to wild-type animals ( Supplementary Fig. 5d ), suggesting that these molecules are not necessary for cold tolerance. Since the insulin-signalling pathway is involved in dauer larva formation, we tested other signalling molecules that are important for dauer larva formation, such as molecular components of transforming growth factor-beta (TGF-β) and steroid hormonal signalling ( Fig. 6a ) [31] . However, we did not observe strong defects in temperature experience-dependent cold tolerance in these mutants ( Fig. 6a ). These genetic experiments suggest that the insulin-signalling pathway is essential for cold tolerance, but that TGF-β and steroid hormone signalling are not essential. In many organisms, including the nematode, the percentage of different fatty acids in the body is important for the formation of cold tolerance [1] . A previous report by Murray et al . [1] demonstrated that the percentage of fatty acids changed depending on the cultivation temperature, which was important for cold tolerance. In addition, Savory et al . [2] showed that FOXO-type transcription factor DAF-16, which is involved in insulin signalling, is important for delta-9 desaturase gene expression, which is important for survival at low temperatures. We therefore measured the fatty acid composition of total lipids in daf-2 /insulin receptor mutants. We found that the fatty acid composition of total lipids was different between wild type and daf-2 mutants ( Supplementary Fig. 6a,b ). These results are consistent with previous reports that DAF-16/FOXO regulates genes involved in lipid production. Insulin is a secretory molecule, and the insulin receptor DAF-2 is expressed in many tissues, such as neurons, muscles and intestine [32] . To investigate tissues where DAF-2 functions in temperature experience-dependent cold tolerance, we tested the cold tolerance of daf-2 animals expressing daf-2cDNA in neurons, intestine or muscles. The tissue-specific rescue experiments revealed that the DAF-2/insulin receptor functions in both intestine and neurons ( Fig. 6b , daf-2(e1370);Ex[unc-14p::daf-2, ges-1p::daf-2] (neuron and intestine)). These results suggest that the insulin-signalling pathway in intestine and neurons is essential for temperature experience-dependent cold tolerance of animals. A recent study has shown that worm intestine itself is highly cold sensitive, and that this tissue plays a central role in ageing and the stress response, in which the cold receptor transient receptor potential (TRP) channel encoded by trpa-1 is essential [33] . We therefore tested the function of trpa-1 and its downstream molecule pkc-2 encoding protein kinase C in cold tolerance. Loss-of-function mutants of trpa-1 and pkc-2 showed normal phenotypes when compared with wild type ( Fig. 6c ). Also, overexpression of the trpa-1 gene in wild-type intestine did not result in an abnormal phenotype ( Fig. 6c (wild type; XuEx601 )). Besides, overexpression of the trpa-1 gene in the daf-2 /insulin receptor mutant did not suppress abnormalities in the daf-2 single mutants ( Fig. 6c ). These results indicate that TRPA-1 signalling in the intestine is independent of cold tolerance signalling. To determine a downstream insulin-signalling pathway for temperature-dependent cold tolerance, we used previous DNA microarray analysis results measuring temperature change-dependent gene expression [34] . We found that mutants of some genes, such as endonuclease ( M60.2 ) and cysteine protease ( cpr-1) , showed abnormal cultivation-dependent cold tolerance ( Fig. 7a ; Supplementary Fig. 5a ). Expression levels of these genes were significantly changed in daf-2 /insulin receptor mutants ( Fig. 7b ; Supplementary Fig. 5b ), indicating that expression of these genes is directly or indirectly regulated downstream of insulin signalling for temperature experience-dependent cold tolerance. 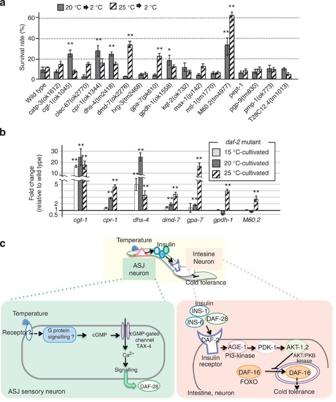Figure 7: Downstream molecules of insulin signalling in cold tolerance. (a) Cold tolerance of mutant animals with impaired genes identified from previous DNA microarray analysis were used to measure temperature change-dependent gene expression34. The gene and encoding protein of the mutants that showed abnormal cold tolerance (with asterisks) are listed in the table inSupplementary Fig. 5a. For each assay,n≥6. Asterisks indicate statistical significance between the wild type and mutant. (b) Results of quantitative PCR of each gene in thedaf-2(e1370)mutant. Each bar represents the relative value of wild type cultivated at each temperature (n=3). Error bars indicate standard error of the mean. Analysis of variance followed by Dunnetpost-hoctest was used for multiple comparisons. *P<0.05; **P<0.01. (c) A molecular and cellular model for temperature experience-inducing cold tolerance. Temperature is detected by the ASJ neuron, in which the trimeric G protein-coupled temperature signal controls insulin secretion. Insulin is received by the intestine and neuron, where insulin signalling regulates gene expression for cold tolerance. We describe here a simple plausible model. Figure 7: Downstream molecules of insulin signalling in cold tolerance. ( a ) Cold tolerance of mutant animals with impaired genes identified from previous DNA microarray analysis were used to measure temperature change-dependent gene expression [34] . The gene and encoding protein of the mutants that showed abnormal cold tolerance (with asterisks) are listed in the table in Supplementary Fig. 5a . For each assay, n ≥6. Asterisks indicate statistical significance between the wild type and mutant. ( b ) Results of quantitative PCR of each gene in the daf-2(e1370) mutant. Each bar represents the relative value of wild type cultivated at each temperature ( n =3). Error bars indicate standard error of the mean. Analysis of variance followed by Dunnet post-hoc test was used for multiple comparisons. * P <0.05; ** P <0.01. ( c ) A molecular and cellular model for temperature experience-inducing cold tolerance. Temperature is detected by the ASJ neuron, in which the trimeric G protein-coupled temperature signal controls insulin secretion. Insulin is received by the intestine and neuron, where insulin signalling regulates gene expression for cold tolerance. We describe here a simple plausible model. Full size image Because cold tolerance can be overwritten within 2–3 h after the cultivation temperature is altered ( Fig. 1f,g ; Supplementary Fig. 1d,e ), we examined calcium measurements in the ASJ neurons during longer times by extending the calcium imaging assays to measure points at 30 min to 5 h ( Fig. 3e ). We found that the calcium concentration was at its maximum at 30 min after the temperature changed from 17–23 °C, and was strongly decreased at 1 h. The results of calcium imaging of ASJ neurons over longer time periods after warming ( Fig. 3e ) showed a prolonged response of ASJ neurons to a step in temperature; it is a sustained response to a higher temperature over 30 min, and it is not a short-term transient response to a changing temperature shown in Fig. 3b . This would be expected in a process having long-term effects on cold tolerance. Physiological calcium imaging analysis in this study suggests that ASJ neurons continue to respond to temperature for at least 30 min ( Fig. 3e ). Since the cold tolerance phenotype can be replaced within 2–3 h after changing the cultivation temperature ( Fig. 1f,g ; Supplementary Fig. 1d,e ), ASJ-dependent insulin secretion could continue for 30 min to 1 h. After that, downstream events of insulin signalling, such as gene expression and changing cell metabolism in the intestine and neurons, may determine cold tolerance within 2–3 h. Exploring the mechanisms for temperature habituation of animals is an important challenge in life sciences. The results in this study demonstrated that experience-dependent cold tolerance is regulated by a single sensory neuron, ASJ, known as light and pheromone-sensing neuron. ASJ neurons release insulin, which is received by the intestine and other neurons in C. elegans ( Fig. 7c ). Our genetic and physiological analysis suggested that ASJ sensory neurons secrete insulin molecules that result in decreasing cold tolerance in wild-type animals. Thus, ASJ-dependent insulin signalling acts as a negative regulator of cold tolerance. In contrast, our genetic model described a positive regulator, the DAF-16/FOXO-type transcription factor. Because daf-16 single mutants only showed a partial decrement of cold tolerance after cultivation at 18 °C ( Supplementary Fig. 4b ), we hypothesize that there is additional positive signalling in cold tolerance. As previously reported, DAF-16 regulates the gene expression of the delta-9 desaturase gene, which is important for cold tolerance in many animals, including worms, and impairment of the delta-9 desaturase gene decreases cold tolerance in worms [2] . Based on these data, we propose two plausible models. In the first model, an unidentified temperature-sensing system in the nervous system and/or other tissues controls positive signalling for cold tolerance, although mutant animals with an impaired nervous system have not shown an abnormal decrement of cold tolerance. Alternatively, we can propose another model, where DAF-16 and an unidentified transcription factor could be activated under default conditions without temperature stimuli. This model is consistent with a previous result, where translocation of DAF-16/FOXO between the nucleus and cytoplasm is not observed following cold stimuli [2] , but is observed at ambient temperatures. In either model, ASJ-dependent temperature signalling acts as a gain-controller of cold tolerance through negative regulation of positive signalling for cold tolerance. It is also likely that the cold tolerance is accomplished by more complicated mechanisms, although we describe here a simpler plausible genetic and physiological model ( Fig. 7c ). Molecular physiological systems are mainly conserved from humans to C. elegans , and the systems found in this study can therefore provide a useful model for studying temperature habituation in other animals. Our current work helps explain a complex mechanism for temperature habituation, from stimulus sensing through the neuronal and intestinal reactions that produce temperature tolerance. Statistical analysis All error bars in the figures, including those in the Supplementary Information , indicate standard error of mean. All statistical analyses in the figures, including those in the Supplementary Information , were performed by one-way analysis of variance for multiple comparisons, which were followed by Dunnet post-hoc tests. All single asterisk (*) and double asterisk (**) in the figures indicate P <0.05 and P <0.01, respectively. P indicates probability. Molecular biology trx-1p::tax-4 cDNA (pTOM4) , str-3p::tax-4 cDNA (pTOM3) and ceh-36p::tax-4 cDNA (pTOM10) used in Fig. 2e include tax-4 cDNA that was PCR amplified from pDEST- tax-4cDNA (a gift from Dr Iino) [35] and the 3′-untranslated region of unc-54 . In addition, pTOM4 includes the ASJ-specific trx-1 promoter (1.0 kb) [36] , which was from pQZ37 trx-1p::ICE (a gift from Dr Alcedo). pTOM3 includes the ASI-specific str-3 promoter (3.1 kb) from pQZ36 ( str-3p::GFP , a gift from Dr Alcedo). pTOM10 includes the AWC-specific ceh-36 promoter (368 bp) from pAK203. daf-28 cDNA inserted into pUC57 was purchased from GenScript, a DNA synthesizing outsource service company. The trx-1 promoter of trx-1p::daf-28 cDNA (pTOM6), the str-3 promoter of str-3p::daf-28 cDNA (pTOM7) and the ceh-36 promoter of ceh-36p::daf-28 cDNA (pTOM8) used the same fragment as mentioned above. To construct DAF-28 fused with fluorescent protein ( trx-1p::daf-28::dsRedm (pOTA11)), we deleted the stop codon of daf-28 cDNA from pTOM6 by site-directed mutagenesis, and then the DsRed monomer DNA was inserted between the daf-28 cDNA and the 3′-untranslated region. trx-1p::snb-1::VENUS (pOTA5) was replaced by the trx-1 promoter from the promoter region of pTAN93 ( glr-3p::snb-1::VENUS ) [37] . trx-1p::yc3.60 was constructed from 1.0 kb trx-1p and the yc3.60 gene derived from pSAS309 ( gcy-8p::yc3.60 ) [17] , [38] . daf-2 cDNA ( Pdpy30-daf-2cDNA ) was provided by Dr Iino and Dr Tomioka. For the construction of unc-14p::daf-2cDNA or ges-1p::daf-2cDNA , the PCR-amplified fragment of daf-2 cDNA was inserted into each plasmid including a 1.5-kb unc-14 promoter (from plasmid pTTu14p) [39] or a 3.3 kb ges-1 promoter (from plasmid pKDK66) [17] . PCR-amplified fragments were verified by sequencing. Temperature experience-inducing cold tolerance assay Uncrowded and well-fed animals were used for the cold tolerance assay. Two adult animals were placed on a 6-cm plate containing 14 ml of nematode growth medium (NGM) with 2% (w/v) agar, on which Escherichia coli OP50 was seeded; the adult animals were transferred to the outside of plate after 8-12 h; the progeny were cultured for about 144–150 h at 15 °C, 85–90 h at 20 °C or 60–65 h at 25 °C. Approximately 70–150 animals were placed on a plate. The plates containing fully matured but not old adult animals were transferred to 2 °C ( Figs 2 , 3 , 4 , 5 , 6 , 7 ; Supplementary Figs 3–5 ) or to a designated cold temperature ( Fig. 1 ; Supplementary Fig. 1 ) in a refrigerated cabinet (MIR-553, Sanyo, Japan). Temperature was monitored by both a digital thermometer and a mercury thermometer. After 48 h ( Figs 2 , 3 , 4 , 5 , 6 , 7 ; Supplementary Figs 3–5 ) or a designated time ( Fig. 1 ; Supplementary Fig. 1 ), the plates were transferred to room temperature (22–24 °C), and the living or dead animals on the plate were counted. In vivo calcium imaging In vivo calcium imaging was performed essentially according to previous reports [17] , [38] . Well-fed animals expressing yellow cameleon 3.60 driven by the trx-1 promoter, trx-1p::yc3.60 (pTOM13), were used for calcium imaging. Animals were glued onto a 2% (w/v) agar pad on glass, immersed in M9 buffer and covered by a cover glass. For long time calcium imaging ( Fig. 3e ), animals were immobilized by 0.1-μm diameter polystyrene microspheres (Polysciences 00876–15, 2.5–5% w/v suspension) on 10% (w/v) agar pads on glass, and covered by a cover glass. After long time calcium imaging, animals were checked to still be alive. Sample preparation was completed within 3 min. The sample was then placed onto a Peltier-based thermocontroller (Tokai Hit, Japan) on the stage of an Olympus IX81 at the initial imaging temperature for 2 min, and fluorescence was introduced into a Dual-View optics system (Molecular Devices, USA). Fluorescence images of donor and acceptor fluorescent protein in yellow cameleon were simultaneously captured using an EM-CCD camera EVOLVE512 (Photometrics, USA). Images were taken with a 100-ms exposure time with 1 × 1 binning. The temperature on the agar pad was monitored by a thermometer system, MATS-5500RA-KY (Tokai Hit). For each imaging experiment, fluorescence intensities were measured using the MetaMorph image analysis system (Molecular Device). Relative changes in intracellular calcium concentration were measured as the change in the acceptor/donor fluorescence ratio of yellow cameleon protein (ratio change). All band pass filters for experiments using yellow cameleon were according to previous reports [17] . Germline transformation Germline transformations were essentially performed as described previously [40] . Germline transformations were performed with co-injection mixes consisting of experimental DNA at various concentrations (5–50 ng μl −1 ) and pKDK66 ges-1p::nls-gfp (50 ng μl −1 ), pNAS88 ges-1p::nls-tag rfp (50 ng μl −1 ), or pRF4 rol-6gf as a transgenic marker [41] . Fatty acid composition Lipids were extracted from synchronized cultures of young adults and transmethylated as described previously [1] . Fatty acid methyl esters were analyzed by gas–liquid chromatography and identified by comparing peak retention times with authentic standards. Fatty acid compositions are presented on a percentage weight basis. Quantitative PCR analysis Wild–type animals and daf-2 mutants were individually synchronized at 15 °C. Animals were transferred to 20 or 25 °C, after cultivation at 15 °C for 5 days until they passed the L1–L3 larval stage, because daf-2 mutants show a constitutive dauer larva formation phenotype at 25 °C. Messenger RNA was isolated using the RNeasy kit (Qiagen). The isolated messenger RNA (100 ng) was reverse-transcribed to cDNA using the iScript Advanced cDNA Synthesis kit for RT-PCR (Bio–Rad). Quantitative PCR was performed using primers specific to the genes, Sso Fast EvaGreen Supermix (Bio–Rad) and a DNA Engine Peltier Thermal Cycler–CFX96 (Bio–Rad). Triplicate samples of each dilution were used for quantitative PCR. The average expression of each gene was normalized to that of the house–keeping gene lmn-1 as a reference [34] . The following sets of primers were used for the detection of cgt-1 ; 5′-GCGATTTTTATGAGACCCGATG-3′ and 5′-CGAACATACAACGCCGAGAA-3′, cpr-1 ; 5′-AGCTGGATGCAAACCATACC-3′ and 5′-GGAACAGCGTAGGCAGAGAC-3′, dhs-4 ; 5′-CTTCGATGTTTGACGCCACT-3′ and 5′-CGACCATTGCCTGAGCTTT-3′, dmd-7; 5′-AACGCGAACAGCTAAATGGA-3′ and 5′-GCGTGCCCTTTCAGTACAAC-3′, gpa-7 ; 5′-TCGACGCAGCAATGAATACC-3′ and 5′-TGCCCTCCAACATCTATCACTC-3′, gpdh-1; 5′-GGGTGACAACGGATTATGAGG-3′ and 5′-CCGACGGAACTTGGGTAGAA-3′, M60.2 ; 5′-AAGAAGAGCCCAGACCACGA-3′ and 5′-CATCCGAGGCAATGAAGTTGT-3′. Laser ablation experiments Laser ablation experiments were performed essentially according to previous reports [5] , [6] . ASJ neurons were killed in anesthetized wild-type animals at the L2–3 stage using a Micropoint system laser microbeam (Photonic Instruments, USA). After laser operation, each animal that had been grown at 20 °C to an adult stage on the Nematode growth media (NGM) plate with sufficient food, E. coli OP50, was tested for cold tolerance at 2 °C for 48 h. RNA interference The C. elegans RNA interference (RNAi) library, which had originally been established by Dr Ahringer, was purchased from Source BioScience [42] and used for all RNAi analyses in this study. The feeding RNAi protocol was performed as described [43] . The eri-1; lin-15B strain was [44] , [45] used as a neuron-sensitized strain for RNAi experiments. Confocal microscopy analysis Preparation of samples was according to the following procedure: a 2% (w/v) agarose gel on a micro slide glass was covered with 10 μl of 100-mM NaN 3 and then a few adult worms were placed on the gel. Finally, the gel was covered by glass. Fluorescent images were analyzed by confocal laser microscopy (FV1000-IX81 with GaAsP photomultiplier tubes, Olympus), using FV10-ASW software (Olympus). How to cite this article: Ohta, A. et al . Light and pheromone-sensing neurons regulates cold habituation through insulin signalling in Caenorhabditis elegans . Nat. Commun. 5:4412 doi: 10.1038/ncomms5412 (2014).